A unifying model for Neoproterozoic–Palaeozoic exceptional fossil preservation through pyritization and carbonaceous compression Soft-tissue fossils capture exquisite biological detail and provide our clearest views onto the rise of animals across the Ediacaran–Cambrian transition. The processes contributing to fossilization of soft tissues, however, have long been a subject of debate. The Ediacaran Gaojiashan biota displays soft-tissue preservational styles ranging from pervasive pyritization to carbonaceous compression, and thus provides an excellent opportunity to dissect the relationships between these taphonomic pathways. Here geochemical analyses of the Gaojiashan fossil Conotubus hemiannulatus show that pyrite precipitation was fuelled by the degradation of labile tissues through bacterial sulfate reduction (BSR). Pyritization initiated with nucleation on recalcitrant tube walls, proceeded centripetally, decelerated with exhaustion of labile tissues and possibly continued beneath the BSR zone. We propose that pyritization and kerogenization are regulated principally by placement and duration of the decaying organism in different microbial zones of the sediment column, which hinge on post-burial sedimentation rate and/or microbial zone thickness. Soft-tissue fossils in the geological record are rare relative to the profusion of shelly hard parts. While shelly organisms produce mineralized structures in vivo , soft tissues require authigenic mineralization to enter the fossil record. The factors contributing to soft-tissue mineralization can be partitioned into two distinct but complementary categories: those that facilitate and those that drive preservation. Facilitating factors are typically palaeoenvironmental in nature, serving to chemically or mechanically delay or inhibit aggressive aerobic degradation (noted in ref. 1 as ‘distal environmental and diagenetic conditions’). While independently invoked as responsible for soft-tissue preservation, facilitating factors are neither mutually exclusive nor sufficient to guarantee fossilization. These conditions can only enable soft-tissue preservation, because delaying degradation is only part of the preservational puzzle. Driving factors refer to constructive mineralization processes that replicate or stabilize soft tissues (‘proximal causes’ of ref. 1 ), ensuring their survivability through geological time and diagenetic alteration. Counterintuitively, many mineralization processes are dependent on microbially mediated degradation to provide and locally concentrate necessary chemical constituents. Each case of soft-tissue preservation is thus a race between destructive decay and constructive mineralization processes [2] . Superlative fossils occur in a narrow window where neither degradation obliterates nor mineralization overprints important biological details, a scenario contingent on both appropriate settings and rapid stabilization processes. Spanning across the Ediacaran–Cambrian transition, when Konservat–Lagerstätten (deposits with exceptional soft-tissue preservation [3] ) are most abundant [4] , [5] , numerous mineralization pathways fulfil the role of soft-tissue stabilizers [6] , [7] . Two of these pathways—Beecher’s Trilobite-type pyritization (three-dimensional pervasive pyritization) and Burgess Shale-type kerogenization (two-dimensional carbonaceous compression)—are particularly important. Pervasive pyritization is commonly facilitated by rapid burial, minimal ambient organic material, periodic or persistent anoxia/dysoxia, reactive iron and sulfate availability, low bioturbation and bacterial sulfate reduction (BSR)-mediated decay [1] , [8] , [9] , [10] , [11] , [12] , [13] , [14] (BSR: CH 3 COO − +SO 4 2– →2 HCO 3 – +HS – ). By and large, kerogenization has been attributed to many of the same facilitating conditions, mostly related to rapid burial into anoxic/dysoxic palaeoenvironments [15] . While numerous other palaeoenvironmental and diagenetic considerations have been invoked for kerogenization, such as interactions with clays [6] , [16] or ferrous iron [17] , high alkalinity [15] , [18] and oxidant restriction (that is, lack of sulfate for BSR) through early diagenetic sealing [18] (though see also ref. 19 ), the common association of kerogenized fossils with pyrite [1] , [6] , [12] , [16] , [20] , [21] , [22] , [23] , [24] bolsters the interrelationship of these taphonomic processes. Fossils in the late Ediacaran (~551–541 Ma) Gaojiashan Lagerstätte illustrate a preservational gradient from pervasive pyritization to compressed kerogenization [1] , including three-dimensional pervasive pyritization, incomplete pyritization and carbonaceous compression with associated pyritization. As such, this Lagerstätte offers an opportunity to establish a comprehensive taphonomic model marrying these pathways. To this end, we geochemically investigate the abundant Gaojiashan fossil Conotubus hemiannulatus , which shows preservation in each of these taphonomic styles. Our data form the basis for the proposed unifying model, which invokes sedimentation rate, and thus time the decaying carcass spends in specific microbial zones, to regulate taphonomic styles along the pyritization–kerogenization gradient. General taphonomic observations Among hundreds of Conotubus specimens examined in this study, ~80% are preserved three-dimensionally through complete or incomplete pyritization ( Fig. 1a,b ), with the remaining preserved through two-dimensional kerogenization [1] ( Fig. 1c ). Pervasively pyritized Conotubus specimens possess secondary cracks filled with calcite cements, and thin rinds (<20 μm) of iron oxide along these cracks ( Figs 2g , 3c and 4e ). Viewed in longitudinal and transverse cross-sections ( Figs 2a , 3a and 4b ), these specimens show a bimodal size distribution of pyrite crystals. Generally, a micrometric size class of crystals ranges from ~10 to ~250 μm, and a millimetric size class of crystals ranges from ~800 μm to a few mm. Micrometric pyrite crystals are mainly found at the outer edge of the fossil ( Figs 2a and 3a ) and sometimes along non-continuous central voids ( Fig. 3a ) or fractures ( Figs 2a and 4b ), whereas millimetric pyrite crystals comprise the bulk of the tube interior ( Fig. 2a ). In some cases, millimetric crystals appear to be amalgamations of micrometric crystals ( Fig. 3a ). In others, millimetric crystals appear to have subtle textural variations along their outer edges, possibly indicative of later overgrowth ( Fig. 2b,c ). 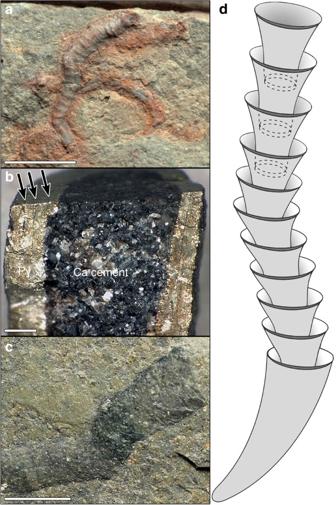Figure 1: Taphonomic representations ofConotubus hemiannulatus. (a) Pervasively pyritized (rusty weathered colour)Conotubuson bedding plane. Scale bar, 5 mm. (b) Longitudinally fracturedConotubusspecimen showing carbonate cement infill (labelled Ca cement), with pyritized (labelled Py) nested funnel walls visible (arrows). Scale bar, 1 mm. (c) Specimen ofConotubuspreserved as two-dimensional carbonaceous compressions with aluminosilicate coating. Scale bar, 5 mm. (d) Interpretive schematic ofConotubusshowing flexible, funnel-in-funnel tube structure and morphology. Figures inb,care reproduced with permission from Elsevier (modified from ref.28and ref.1, respectively). Figure 1: Taphonomic representations of Conotubus hemiannulatus . ( a ) Pervasively pyritized (rusty weathered colour) Conotubus on bedding plane. Scale bar, 5 mm. ( b ) Longitudinally fractured Conotubus specimen showing carbonate cement infill (labelled Ca cement), with pyritized (labelled Py) nested funnel walls visible (arrows). Scale bar, 1 mm. ( c ) Specimen of Conotubus preserved as two-dimensional carbonaceous compressions with aluminosilicate coating. Scale bar, 5 mm. ( d ) Interpretive schematic of Conotubus showing flexible, funnel-in-funnel tube structure and morphology. Figures in b , c are reproduced with permission from Elsevier (modified from ref. 28 and ref. 1 , respectively). 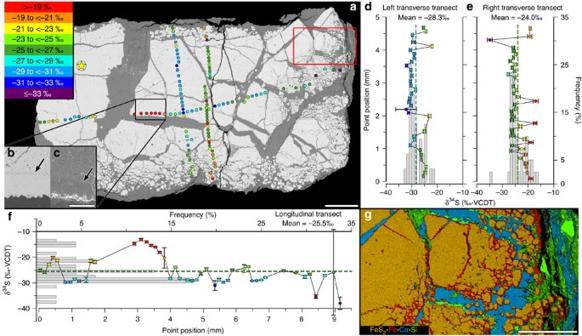Figure 2: SEM/EDS and SIMS δ34SPYdata forConotubusspecimen GJS-Cono001. (a) Backscatter Z-contrast electron micrograph montage of longitudinal section, with all SIMS spots (circles) plotted at analysis location. Microdrilling location for IRMS δ34SPYassessment indicated by star. Point and star colour corresponds to δ34SPYbins shown in upper left key. Scale bar, 1 mm. Insets (b,c) at lower left show higher magnification split-frame of black rectangle region highlighting subtle textural difference associated with pyrite overgrowth (arrows in each panel); backscatter electron (b) and secondary electron (c) images. Scale bar, 250 μm. (d–f) SIMS transects, with dashed lines indicating mean values and histograms showing frequency of points by 1‰ bins. Note generalized U-shaped profile ind(left transect), with higher values towards fossil edges and lower values centrally located. To show precision of each 10-cycle point sample mean, error bars mark±1 standard error. These errors do not include the analytical uncertainties of the Balmat pyrite standard, which are relatively small. (g) Energy-dispersive X-ray elemental overlay of iron-sulfur (gold), iron but no sulfur (red), calcium (blue) and silicon (green). Map region corresponds to red rectangle ina. Scale bar, 500 μm. Full size image Figure 2: SEM/EDS and SIMS δ 34 S PY data for Conotubus specimen GJS-Cono001. ( a ) Backscatter Z-contrast electron micrograph montage of longitudinal section, with all SIMS spots (circles) plotted at analysis location. Microdrilling location for IRMS δ 34 S PY assessment indicated by star. Point and star colour corresponds to δ 34 S PY bins shown in upper left key. Scale bar, 1 mm. Insets ( b , c ) at lower left show higher magnification split-frame of black rectangle region highlighting subtle textural difference associated with pyrite overgrowth (arrows in each panel); backscatter electron ( b ) and secondary electron ( c ) images. Scale bar, 250 μm. ( d – f ) SIMS transects, with dashed lines indicating mean values and histograms showing frequency of points by 1‰ bins. Note generalized U-shaped profile in d (left transect), with higher values towards fossil edges and lower values centrally located. To show precision of each 10-cycle point sample mean, error bars mark±1 standard error. These errors do not include the analytical uncertainties of the Balmat pyrite standard, which are relatively small. ( g ) Energy-dispersive X-ray elemental overlay of iron-sulfur (gold), iron but no sulfur (red), calcium (blue) and silicon (green). Map region corresponds to red rectangle in a . Scale bar, 500 μm. 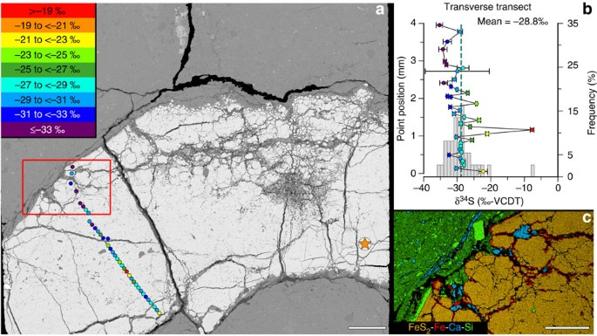Figure 3: SEM/EDS and SIMS δ34SPYdata forConotubusspecimen GJS-Cono002. (a) Backscatter Z-contrast electron micrograph montage of longitudinal section, with all SIMS spots (circles) plotted at analysis location. Microdrilling location for IRMS δ34SPYassessment indicated by star. Point and star colour corresponds to δ34SPYbins shown in upper left key. Scale bar, 1 mm. (b) SIMS transect, with dashed line indicating mean value, and histogram showing frequency of points by 1‰ bins. To show precision of each 10-cycle point sample mean, error bars mark±1 s.e. These errors do not include the analytical uncertainties of the Balmat pyrite standard, which are relatively small. (c) EDS elemental overlay of iron-sulfur (gold), iron but no sulfur (red), calcium (blue) and silicon (green). Map region corresponds to red rectangle ina. Scale bar, 500 μm. Full size image Figure 3: SEM/EDS and SIMS δ 34 S PY data for Conotubus specimen GJS-Cono002. ( a ) Backscatter Z-contrast electron micrograph montage of longitudinal section, with all SIMS spots (circles) plotted at analysis location. Microdrilling location for IRMS δ 34 S PY assessment indicated by star. Point and star colour corresponds to δ 34 S PY bins shown in upper left key. Scale bar, 1 mm. ( b ) SIMS transect, with dashed line indicating mean value, and histogram showing frequency of points by 1‰ bins. To show precision of each 10-cycle point sample mean, error bars mark±1 s.e. These errors do not include the analytical uncertainties of the Balmat pyrite standard, which are relatively small. ( c ) EDS elemental overlay of iron-sulfur (gold), iron but no sulfur (red), calcium (blue) and silicon (green). Map region corresponds to red rectangle in a . Scale bar, 500 μm. 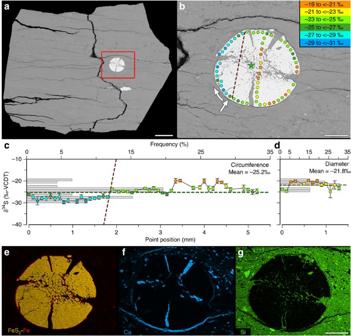Figure 4: SEM/EDS and δ34SPYdata forConotubusspecimen GJS-Cono003. (a,b) Backscatter Z-contrast electron micrograph montage of transverse section, with all SIMS spots (circles) plotted at analysis location. Microdrilling for IRMS δ34SPYwas made on the reverse side of the specimen at a location corresponding to the star. Point and star colour corresponds to δ34SPYbins shown in upper right key. Scale bar ina, 2 mm, inb, 500 μm. (c,d) SIMS circumference and diameter transects, respectively, with dashed lines indicating mean values, and histograms showing frequency of points by 1‰ bins. Circumference δ34SPYplot follows clockwise from straight arrow inb. Using dashed red line inbas a reference, note slight separation of δ34SPYvalues: higher δ34SPYvalues to the right and lower δ34SPYvalues to the left of the dashed line inb. Diameter δ34SPYplot follows top-to-bottom. To show the precision of each 10-cycle point sample mean, error bars mark±1 s.e. These errors do not include the analytical uncertainties of the Balmat pyrite standard, which are relatively small. (e–g) EDS elemental overlay of iron-sulfur (gold), iron but no sulfur (red), calcium (blue) and silicon (green). Map region corresponds to red rectangle ina. Scale bar ingis 500 μm, applicable foreandf. Full size image Figure 4: SEM/EDS and δ 34 S PY data for Conotubus specimen GJS-Cono003. ( a , b ) Backscatter Z-contrast electron micrograph montage of transverse section, with all SIMS spots (circles) plotted at analysis location. Microdrilling for IRMS δ 34 S PY was made on the reverse side of the specimen at a location corresponding to the star. Point and star colour corresponds to δ 34 S PY bins shown in upper right key. Scale bar in a , 2 mm, in b , 500 μm. ( c , d ) SIMS circumference and diameter transects, respectively, with dashed lines indicating mean values, and histograms showing frequency of points by 1‰ bins. Circumference δ 34 S PY plot follows clockwise from straight arrow in b . Using dashed red line in b as a reference, note slight separation of δ 34 S PY values: higher δ 34 S PY values to the right and lower δ 34 S PY values to the left of the dashed line in b . Diameter δ 34 S PY plot follows top-to-bottom. To show the precision of each 10-cycle point sample mean, error bars mark±1 s.e. These errors do not include the analytical uncertainties of the Balmat pyrite standard, which are relatively small. ( e – g ) EDS elemental overlay of iron-sulfur (gold), iron but no sulfur (red), calcium (blue) and silicon (green). Map region corresponds to red rectangle in a . Scale bar in g is 500 μm, applicable for e and f . Full size image Sulfur isotopic data Pyrite sulfur isotopic values (δ 34 S PY ), measured using secondary ion mass spectroscopy (SIMS), range between –7.6 and –37.9‰-VCDT ( Supplementary Table 1 and Fig. 2a,d–f ; Fig. 3a,b ; Fig. 4b–d ). Although not a hard-and-fast rule, pyrite with δ 34 S PY values ≥–19‰ tend to be associated with fractures and/or textural variations in the pyritized fossil, which may correspond to later overgrowth (for instance, see adjacent red points in Fig. 2a longitudinal transect positioned just below arrows indicating textural variation in Fig. 2b,c ). Disregarding obvious fracture-associated 34 S-enriched points, the transverse δ 34 S PY transects exhibit a generalized U-shaped profile, with localization of greater values along the tube-wall edges and lower values towards the center of the fossil ( Fig. 2d,e ). This pattern is not discernable in all specimens ( Figs 3b and 4c,d ). Microdrilled pyrite assessed via isotope ratio mass spectroscopy (IRMS) yield δ 34 S PY values broadly similar to mean SIMS values ( Supplementary Table 1 ). Carbonate-associated sulfate sulfur isotopic composition (δ 34 S CAS ) of host rock was assessed at +33.6‰-VCDT ( Supplementary Table 1 ), comparable to contemporaneous units in Oman [25] . Thus, Δ 34 S CAS-PY is appreciably high (ranging from +41.2 to 71.5‰). Carbon and oxygen isotopic data Three-dimensionally but incompletely pyritized Conotubus specimens show an outer rim of pyrite, with multiple generations of compositionally distinct carbonate cements surrounding a central void in the tube interior ( Fig. 5 ). In the only chemically analysed cross-section with this preservational style but representative of other similarly preserved specimens, the outer first generation cements consist of large centripetally terminating calcite crystals, indicating inward carbonate growth from the pyrite rim. The inner second generation cements are zoned rhombohedral crystals, with alternating ultraviolet-luminescent zones of ferroan dolomite and dull zones of dolomite+calcite. Carbon and oxygen isotopic compositions of microlaminae in the host rock and for the two generations of fossil carbonate cements were determined ( Supplementary Table 2 and Fig. 6 ). The mean δ 13 C value of the darker coloured microlaminae (6.1±0.9‰ VPDB) is greater than that of the lighter coloured microlaminae (4.4±1.0‰) with slight overlap in ranges, whereas their mean δ 18 O values are broadly similar (darker microlaminae=–5.4±1.2‰; lighter microlaminae=–5.9±0.3‰) with mostly overlapping ranges. While similar in carbon isotope composition, the cements in the Conotubus tube and the host rock have distinct δ 18 O values. Between fossil-interior cement generations, the outer calcite cements have slightly greater mean δ 13 C and δ 18 O values (δ 13 C=6.1±0.1‰, δ 18 O=–8.2±0.2‰) than the inner dolomite+calcite cements (δ 13 C=5.2±0.4‰, δ 18 O=–9.0±0.2‰). 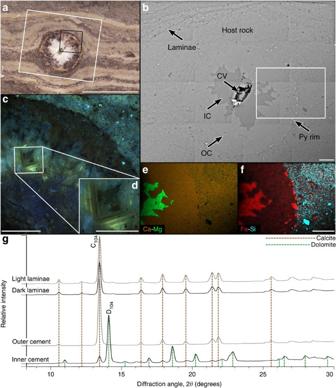Figure 5: Ultraviolet photoluminescence andin situXRD data forConotubusspecimen 1GH2-70A. (a) Overview photomicrograph of transverse slab ofConotubusand surrounding matrix of laminated rock. Note pyrite or iron oxide rim (gold colour), outer carbonate cement (dark colour), inner carbonate cement (light colour) and central void. Scale bar, 10 mm. (b) Backscattered Z-contrast electron micrograph montage of region defined by white rectangle ina. Fine pyrite or iron oxide rim (Py rim) seen as bright discontinuous specks, surrounding carbonate cements (IC: inner cement; OC: outer cement) and central void (CV). Scale bar, 1 mm. (c) Ultraviolet photoluminescence microscopy of black rectangle region ina, showing zoned carbonate crystals in inner cement. Scale bar, 1 mm. Inset (d) shows higher magnification view of white rectangle incfor better detail of crystal zoning. Scale bar, 500 μm. (e,f) EDS elemental maps of white rectangle region inb, with calcium (orange) and magnesium (green) overlay shown ineand iron (red) and silicon (blue) overlay shown inf. Scale bar infis 1 mm, applicable fore. (g)In situXRD patterns of host rock light- and dark-coloured laminae, outer carbonate cement within fossil and inner carbonate cement within fossil. Characteristic peak positions of calcite and dolomite are shown in orange and green vertical dashed lines, respectively. The strongest diffraction peaks from calcite and dolomite are labelled with C104and D104, respectively. Figure 5: Ultraviolet photoluminescence and in situ XRD data for Conotubus specimen 1GH2-70A. ( a ) Overview photomicrograph of transverse slab of Conotubus and surrounding matrix of laminated rock. Note pyrite or iron oxide rim (gold colour), outer carbonate cement (dark colour), inner carbonate cement (light colour) and central void. Scale bar, 10 mm. ( b ) Backscattered Z-contrast electron micrograph montage of region defined by white rectangle in a . Fine pyrite or iron oxide rim (Py rim) seen as bright discontinuous specks, surrounding carbonate cements (IC: inner cement; OC: outer cement) and central void (CV). Scale bar, 1 mm. ( c ) Ultraviolet photoluminescence microscopy of black rectangle region in a , showing zoned carbonate crystals in inner cement. Scale bar, 1 mm. Inset ( d ) shows higher magnification view of white rectangle in c for better detail of crystal zoning. Scale bar, 500 μm. ( e , f ) EDS elemental maps of white rectangle region in b , with calcium (orange) and magnesium (green) overlay shown in e and iron (red) and silicon (blue) overlay shown in f . Scale bar in f is 1 mm, applicable for e . ( g ) In situ XRD patterns of host rock light- and dark-coloured laminae, outer carbonate cement within fossil and inner carbonate cement within fossil. Characteristic peak positions of calcite and dolomite are shown in orange and green vertical dashed lines, respectively. The strongest diffraction peaks from calcite and dolomite are labelled with C 104 and D 104 , respectively. 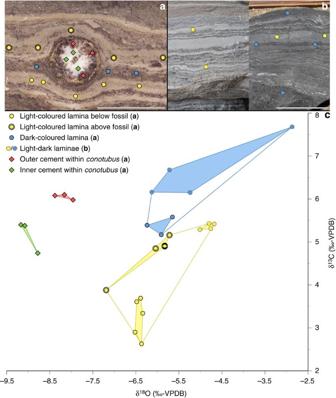Figure 6: Host rock and fossil carbonate IRMS δ13C and δ18O data. (a) Microdrill map of slab 1GH2-70A withConotubusspecimen. Scale bar, 10 mm. (b) Microdrill map of slab (two continuous pieces) withoutConotubusfossils. Scale bar, 50 mm. (c) Cross-plot of all δ13C and δ18O analyses. Convex hulls and nested convex hulls (shaded) show groupings of data by location of microsampling. Yellow points show light-coloured laminae (single circle below fossil and double circle above fossil ina; dashed circle from slab inb). Blue points show dark-coloured laminae (single circle contiguous to fossil ina; dashed circle from slab inb). Red and green diamonds show outer and inner cements ina, respectively. Keys also applicable for microdrill location maps. Full size image Figure 6: Host rock and fossil carbonate IRMS δ 13 C and δ 18 O data. ( a ) Microdrill map of slab 1GH2-70A with Conotubus specimen. Scale bar, 10 mm. ( b ) Microdrill map of slab (two continuous pieces) without Conotubus fossils. Scale bar, 50 mm. ( c ) Cross-plot of all δ 13 C and δ 18 O analyses. Convex hulls and nested convex hulls (shaded) show groupings of data by location of microsampling. Yellow points show light-coloured laminae (single circle below fossil and double circle above fossil in a ; dashed circle from slab in b ). Blue points show dark-coloured laminae (single circle contiguous to fossil in a ; dashed circle from slab in b ). Red and green diamonds show outer and inner cements in a , respectively. Keys also applicable for microdrill location maps. Full size image Compaction Three-dimensional preservation of Conotubus allows an estimate of the compaction ratio of the host sediments. Viewed perpendicular to bedding plane, the calcisiltite/calcilutite microlaminae warp around nearly circular Conotubus tubes ( Figs 4a,b , 5 and 6 ). Measurements of microlaminae surrounding Conotubus tubes in comparison with their thickness extending beyond the fossil yields an estimated sediment compaction ratio of ~1.85:1. Conotubus tubes show negligible compaction, with a major:minor axis ratio of ~1.15:1, although an oblate cross-section may be biological [26] . Previous analyses of pyritized Palaeozoic Lagerstätten suggest rapid burial into anoxic sediments, which in turn reduces bioturbation, impedes organic deterioration and emplaces the decaying carcasses within the sulfidic BSR zone below the oxic-anoxic boundary in the sediment profile. Further, pyritization-conducive sediments typically have low organic carbon content and abundant reactive iron, serving to focus BSR and pyrite precipitation on decaying carcasses [8] , [9] , [13] , [14] , [27] . While the Gaojiashan biota is similar to these younger deposits in that pyritized fossils are found in sediments deposited by rapid burial events [11] , there are some key differences. First, the full pyritization–kerogenization preservational gradient from three-dimensional pervasive pyritization to two-dimensional kerogenized compressions, with intermediate or admixed preservational modes, appears to be unique to the Gaojiashan Lagerstätte. Second, the tubular fossils of the Gaojiashan biota notably do not retain their most labile soft parts [10] , [28] , showing no evidence of the soft-bodied organisms that lived within these tubes. While some sites of pervasive pyritization show glimpses of highly labile soft-tissue preservation, such as pygnogonid and crustacean musculature from the Hünsruck Slate [29] , [30] , pervasive pyritization of Conotubus only captures the three-dimensional exterior morphologies of the tubes. The original histology of Conotubus tubes is unknown. However, they have been interpreted as supportive, refractory tissues, either non-biomineralized or weakly biomineralized [28] . Building upon the Raiswell et al . [31] diffusion–precipitation model for pyritization, we can begin to elucidate the progression of pervasive fossil pyritization and provide insights into early diagenetic conditions responsible for the taphonomic styles observed in the Gaojiashan Lagerstätte. According to this model [31] , the locus of mineralization is controlled by the intersection of two diffusion fields. The first arises as a consequence of BSR, driving sulfide outward into the sediment porewaters. The second originates from sediment sources, carrying reactive iron toward the decaying organic nucleus. The intersection of these two diffusion fronts results in supersaturated porewaters with respect to iron sulfide at some distance from the organic nucleus. The spatial trends in both pyrite crystal morphology and δ 34 S PY values of Conotubus fossils are consistent with centripetal pyrite growth controlled by the diffusion–precipitation dynamics of mineralization [31] . Similar to the formation of pyrite rims around chert nodules [32] and carbonate concretions [8] , [31] , sulfate reducing bacteria (SRB) metabolized a centrally located organic nucleus, in this case the labile tissues of the Conotubus organism, generating an outward diffusion of sulfide. The sulfide meets with an inward-diffusing reactive iron sourced from ambient porewater, forming a reaction front where pyrite-precursor iron monosulfide [33] precipitation occurs. As this process proceeds, the organic nucleus is progressively exhausted, resulting in an inward shift in the reaction front ( Supplementary Fig. 1 ). One complicating issue, however, is that the recalcitrant tube walls of Conotubus would form a barrier to impede but not entirely halt diffusion, resulting in accumulation of sulfide and reactive iron on either side of the tube walls. As such, we must consider another important factor controlling the locus of pyritization: heterogeneous nucleation facilitated by an organic substrate. The individually conserved nested Conotubus tube walls ( Figs 1b and 7b ) may have promoted pyritization by providing a naturally favourable substrate for the initiation of iron sulfide nucleation—an unaccounted-for factor in the traditional model [31] . 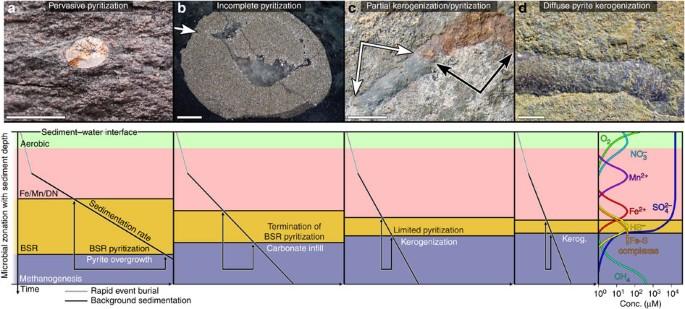Figure 7: Pyritization–kerogenization taphonomic gradient. Fossil examples (a–d, upper panels) and proposed taphonomic model (lower panels) with sedimentary microbial zonation. Diagonal lines track the position of the decaying organisms in the sediment column, and the slope of each line represents sedimentation rate. Grey upper diagonal line corresponds to rapid event burial, and black lower diagonal line corresponds to post-burial sedimentation. Brackets indicate the length of time the decaying organism resides in the BSR zone (gold colour), and experiences BSR-mediated pyrite growth, although pyrite overgrowth may continue into underlying methanogenesis zone (blue colour). From left to right, each diagram indicates a shortened residence time in the BSR zone as compared with the previous panel, which could result from either, or both, changes in post-burial sedimentation rate and BSR zone thickness. (a) Pervasively pyritizedConotubusin transverse cross section. Scale bar, 2.5 mm. Diagram shows initial rapid event deposition, followed by slow post-burial sedimentation. (b) Polished transverse cross-section of pyritizedConotubusshowing carbonate in the center and thin outer lamina (arrow) representing nested tube wall. Scale bar, 1 mm. Corresponding diagram shows increase in post-burial sedimentation rate and reduction in BSR zone thickness, leading to comparatively earlier termination of pyritization. (c) Specimen ofConotubuswith admixed taphonomic mode of pyritization (black arrows) and carbonaceous compression (white arrows). Scale bar, 5 mm. Diagram shows further increase in post-burial sedimentation rate and reduction in BSR zone thickness, yielding partial pyritization and onset of kerogenization once carcass exits BSR zone. (d) Specimen ofConotubuspreserved via complete kerogenization with diffuse pyrite. Scale bar, 5 mm. Diagram shows highest post-burial sedimentation rate and thinnest BSR zone, with limited pyritization, and earliest onset of kerogenization. Relative abundances of chemical species at right follows that of refs47,48after ref67. Fe–S complexes curve shows possible continued pyrite overgrowth from downward diffusion of HS–/Fe2+. Figures ina–dare reproduced with permission from Elsevier (modified from ref.1and ref.28). Figure 7: Pyritization–kerogenization taphonomic gradient. Fossil examples ( a – d , upper panels) and proposed taphonomic model (lower panels) with sedimentary microbial zonation. Diagonal lines track the position of the decaying organisms in the sediment column, and the slope of each line represents sedimentation rate. Grey upper diagonal line corresponds to rapid event burial, and black lower diagonal line corresponds to post-burial sedimentation. Brackets indicate the length of time the decaying organism resides in the BSR zone (gold colour), and experiences BSR-mediated pyrite growth, although pyrite overgrowth may continue into underlying methanogenesis zone (blue colour). From left to right, each diagram indicates a shortened residence time in the BSR zone as compared with the previous panel, which could result from either, or both, changes in post-burial sedimentation rate and BSR zone thickness. ( a ) Pervasively pyritized Conotubus in transverse cross section. Scale bar, 2.5 mm. Diagram shows initial rapid event deposition, followed by slow post-burial sedimentation. ( b ) Polished transverse cross-section of pyritized Conotubus showing carbonate in the center and thin outer lamina (arrow) representing nested tube wall. Scale bar, 1 mm. Corresponding diagram shows increase in post-burial sedimentation rate and reduction in BSR zone thickness, leading to comparatively earlier termination of pyritization. ( c ) Specimen of Conotubus with admixed taphonomic mode of pyritization (black arrows) and carbonaceous compression (white arrows). Scale bar, 5 mm. Diagram shows further increase in post-burial sedimentation rate and reduction in BSR zone thickness, yielding partial pyritization and onset of kerogenization once carcass exits BSR zone. ( d ) Specimen of Conotubus preserved via complete kerogenization with diffuse pyrite. Scale bar, 5 mm. Diagram shows highest post-burial sedimentation rate and thinnest BSR zone, with limited pyritization, and earliest onset of kerogenization. Relative abundances of chemical species at right follows that of refs 47 , 48 after ref 67 . Fe–S complexes curve shows possible continued pyrite overgrowth from downward diffusion of HS – /Fe 2+ . Figures in a – d are reproduced with permission from Elsevier (modified from ref. 1 and ref. 28 ). Full size image The ability of an organic substrate, such as the tube walls, to promote mineralization can be readily justified within the constructs of classical nucleation theory. For a cube-shaped nucleus, the relationship between the free energy barrier opposing the formation of a stable nucleus in solution (homogeneous case) and on a foreign substrate is: , where α hom and α het are the interfacial energies of the homogeneous and heterogeneous nuclei. Although α het depends on the balance between the liquid-nucleus, liquid-substrate and substrate-nucleus interfacial tensions, a simple analysis shows that if α hom ≈ α het , the free energy barrier opposing nucleation at a surface is reduced to half of the homogeneous barrier. As nucleation rate shows an exponential dependence on Δ G *, this translates into a substantial increase in the rate of surface nucleation. Indeed, nucleation rates depend strongly on the chemical nature and physical structure of the organic interface. For instance, NH 3 + terminated surfaces can be completely passive to the formation of amorphous SiO 2 ; however, under identical conditions, NH 3 + /COO – surfaces promote SiO 2 deposition to the extent that the organic may be coated by a nearly-coherent nanoscale layer of amorphous material within a few hours [34] . Moreover, as evidenced by calcite nucleation on polysaccharide matrices [35] , significant variations in the surface nucleation rate may occur between biopolymers with similar functionalities, with the specific order of substrate preference depending chiefly on supersaturation. During the earliest stages of microbially induced degradation, when nucleation sites on the tube surface are most abundant, pyritization is dominated by precipitation of abundant micrometric crystals as are observed at the outer edges of the Conotubus specimens. The size and location of the crystallites indicates that the organic tube-wall surface likely plays a role in directing the onset of nucleation, and that the pyrite supersaturation state, σ , was relatively high as compared with the later stages of mineralization when pyritization proceeds through coarsening of existing crystals rather than formation of new crystals. This interpretation is supported by the nucleation rate equation, , where A is a pre-exponential constant (whose units represent the number of molecules attaching to a critically-sized nucleus per unit time and surface area), B is a constant that describes the shape of the nucleus, T is temperature, k B is the Boltzmann constant, Δ G* is free energy matching the thermodynamic barrier opposing nucleation and σ is supersaturation . This equation shows that an increase in supersaturation state generally results in a higher number of nuclei per unit area of substrate or volume of solution in the case of homogeneous nucleation. As compared with any soft body tissues of the Conotubus organism, the tube walls must have provided the most chemically favourable nucleation sites for initiation of pyrite growth. Pyrite crystals in these regions are isotopically heavier (δ 34 S PY typically >–25‰; Fig. 2a,d,e ) than those in the tube interior, indicating a progressive decline in BSR rate throughout the pyritization process and corresponding relaxation in diffusion-limited sulfate availability. The inferred sulfate limitation in initial pyritization may seem contradictory to the high Δ 34 S CAS-PY values ( Supplementary Note 1 ). However, oxidative recycling of sulfide and oxidation of detrital pyrite entrained in microturbidites [14] likely supplied 34 S-depleted sulfate for pyritization, thereby contributing to the high Δ 34 S CAS-PY values. As BSR continues over time, labile tissues are diminished and BSR necessarily slows because of decreasing availability of metabolizable organic carbon rather than sulfate exhaustion or deep burial, which would instead yield a shift towards higher δ 34 S PY values. As a result of slowed BSR, sulfide production rate would drop, supersaturation levels with respect to iron sulfide would decrease and nucleation would be disfavoured. Thus, iron sulfide precipitation is focused on overgrowing existing crystals, leading to the formation of millimetric crystals. During this shift, δ 34 S PY values would decrease as the BSR system switches from sulfate limitation to organic limitation. The expected result is a U-shaped δ 34 S PY profile as observed in some specimens ( Fig. 2d,e ), although this profile can be obscured by pyrite overgrowth (see Discussion below). From the understanding of how the pyritization process proceeds and expectations for resultant sulfur isotopic trends ( Supplementary Note 1 ), we can then shift our focus to resolving the geochemical constraints for pervasive pyritization. With the first dissociation constant of H 2 S at 1.05 × 10 −7 ( K 1 =[H + ][HS − ]/[H 2 S]) and seawater pH typically constrained to ~7.5–8.5, HS – is the dominant dissolved sulfide species. Thus, we can write the precipitation of pyrite as Fe 2+ +S 0 +HS – →FeS 2 +H + , such that the equilibrium solubility product for pyrite is given as K sp =[Fe 2+ ][HS − ]/10 −pH =10 −16.35 (ref. 36 ). With activity coefficients for HS – and Fe 2+ in seawater at 0.67 and 0.26 (ref. 37 ), we can then calculate the apparent solubility product for pyrite as at the low end of normal seawater pH. As such, given the Raiswell et al . [31] model assumption of the estimated ratio of reservoir concentrations ( C 0 ) of sulfur to iron, C S 0 : C Fe 0 <0.1 (that is, [Fe 2+ ]≥10 × [HS – ]), for localized pyrite formation at the site of decay [31] , reactive iron must be greater than approximately 9 × 10 −12 M to drive pyrite precipitation, well below modern observations of anoxic sediments at<10 −4 M (refs 8 , 31 ). Because the majority of the fossils in the Gaojiashan Lagerstätte exhibit three-dimensional pervasive pyritization [1] , we can surmise an excess of available sediment/porewater reactive iron. Assuming a decay constant of 0.1–1.0 per year (reported for organic decay in marine sediments [38] ) and an organic nucleus radius of 0.1–1.0 cm (appropriate for Conotubus with a maximum diameter of 1.2 cm (ref. 28 )), porewater dissolved sulfide concentrations of <10 −4 M are required for soft tissue pyritization ( Fig. 3 in ref. 31 ). As localized pyritization of highly labile tissues occurs when C S 0 : C Fe 0 <0.1 (ref. 31 ), Fe 2+ content in porewater may have been up to 10 −3 M. We can thus reasonably constrain porewater Fe 2+ content in Gaojiashan sediments between 9 × 10 −12 M and 10 −3 M, justified by the lack of labile soft-tissue pyritization in this Lagerstätte. In incompletely pyritized but three-dimensional Conotubus tubes, alkalinity generated during BSR ( Supplementary Table 3 ) and bacterial Fe(III) reduction (BFeR: CH 3 COO − +8 Fe(OH) 3 →2 HCO 3 − +8 Fe 2+ +15 OH – +5 H 2 O) could contribute to carbonate infill assuming appropriately basic microenvironmental pH levels to facilitate calcite precipitation [32] , [39] . While similar relatively heavy δ 13 C values of host rock and fossil cement render BSR- or BFeR-sourced bicarbonate as insignificant contributors, dissolved sulfide is observed to enhance crystallization of calcite and dolomite [40] , possibly contributing to early calcite cementation. In addition, SRB exopolysaccharides commonly incorporate metal cations (such as Mg and Fe), which could facilitate precipitation of high-Mg calcite and ankerite [41] . The ~2‰ difference between carbonate cement δ 18 O values within the Conotubus specimen and host carbonates, but broadly similar δ 13 C values ( Fig. 6c ), suggest that the cements may have been slightly influenced by diagenetic fluids without significant alteration of carbon isotopic composition. Slightly lower δ 18 O and δ 13 C values in the inner versus outer cements indicates a stronger influence of diagenetic fluids on the inner cementation, consistent with petrographic evidence showing a later origin than the outer cements. The relatively small isotopic difference between the cements and sedimentary matrix suggests that carbonate cementation may have occurred shortly after the cessation of pyritization, playing a constructive preservational role by enhancing the rigidity of partially pyritized tubes before sediment compaction. While we have established that both pervasive and incomplete pyritization must have predated sediment compaction based on warping host rock microlaminae encasing the Conotubus fossils, we can further constrain the duration of the pyritization process. To do so, we must consider requisite levels of sulfate, reactive iron and metabolizable organic material. On the basis of the size of Conotubus specimens, with a maximum diameter of 12 mm and length of 3–80 mm (ref. 28 ), the amount of sulfate required for complete pyritization will follow , where V is the volume of the Conotubus tube, ρ is the density of pyrite (≈5 g per cm 3 ) and M pyrite is the molar mass of pyrite (≈ 120 g mol −1 ). Using V = π * r 2 * l for the volume of a cylinder, with Conotubus radius ( r ) and length ( l ) simplified as 5 and 40 mm, the total sulfate required is 0.26 moles. The amount of reactive iron needed is 0.13 moles. The amount of organic carbon needed varies by the electron donor compound used (largely fermentative end products; Supplementary Table 3 ). For simplicity, we use BSR of acetate, which, in accordance with the above constraints, requires 0.52 moles of organic C. If we then assume that the interior volume of Conotubus tube is completely full of soft tissue (an overestimate), with a nested tube-wall thickness of 1 mm ( Fig. 1b ), the volume of soft tissue that contains metabolizable organic material using the same dimensions as above is ~2 cm 3 . Assuming that the soft tissue was pure amorphous carbon (density=~1.8 g cm −3 ), 0.52 moles would occupy a volume of ~3.5 cm 3 , a substantially larger volume than is available within the Conotubus tube. As such, given realistic carbon contents in animal tissues, we can deduce that there is a deficit of endogenous carbon to account for the volume of pyrite precipitated—which is clearly problematic, but disregarded for now and revisited in our model description below. On the basis of these calculations and high-end rates of sulfate reduction in Ediacaran sediments (6.935 mmol cm −3 per year according to ref. 42 , with pervasive anoxic conditions and higher metabolizability of organics before the evolution of vascular plants [32] , [42] , [43] , [44] ), we can calculate an approximate timeframe for generating sufficient HS – to pervasively pyritize a Conotubus tube with a 3.14 cm 3 total volume. If the 0.26 moles of SO 4 2− is derived entirely endogenously within a Conotubus tube, a total of 82.8 mmol HS – per cm 3 is required for pyritizing the full volume of the tube. At a rate of 6.935 mmol cm −3 per year, a total of ~12 years would be required to generate enough HS – for pyritization. Even at modern rates of sulfate reduction, such as measured rates of 0.1 mmol cm −3 per year (ref. 45 ), this yields 828 years to generate enough HS – for pyritization of moderately sized Conotubus tubes. The decaying organism is a BSR hotspot, which should pull in both SO 4 2– and Fe 2+ from the surrounding microenvironment (as opposed to assumed steady-state equilibrium [31] ), thus these cited bulk-sediment rates may overestimate the pyritization time. It is important to note, however, that these estimates assume that HS – is: (1) a rate-limiting factor for pyrite precipitation and (2) entirely derived from BSR in and around the decaying Conotubus organism in the BSR zone. As discussed below, these assumptions may not be valid. From these and previously reported observations [1] , the data presented herein allow for a pragmatic approach to consider the timing, processes, and interrelationship of pyritization and kerogenization. First, the pyritization process is likely initiated in the BSR zone in the sediment column. The sediment column typically consists of an aerobic respiration zone just beneath the water–sediment interface, followed by an anaerobic zone with nitrate, manganese and iron reduction, then the BSR zone, and finally the methanogenesis zone at depth [46] ( Fig. 7 ). For fossil pyritization to occur in the BSR zone, factors directly responsible for BSR-mediated pyrite mineralization—the availability of sulfate, reactive iron, metabolizable organic material and positioning of the carcass within the BSR zone—must overlap with commonly invoked facilitating conditions such as rapid sedimentation and burial, low bioturbation and sediment anoxia. These factors are intimately related. For example, sedimentation rate influences the availability of reactive iron, sulfate and organic carbon in the sediments, thus controlling the thickness of the BSR zone and ultimately how much time the decaying carcass spends here. Because sedimentation rate plays such an important role, we propose a unifying model in which sedimentation rate was the primary factor controlling the pyritization–kerogenization gradient as observed in the Gaojiashan biota ( Fig. 7 ). To help explain the model, we focus on four representative preservational styles along the pyritization–kerogenization gradient: (1) pervasive pyritization, (2) incomplete three-dimensional pyritization, (3) partial kerogenization with abundant pyrite association and (4) kerogenization with limited or highly diffuse pyrite association. For complete pyritization ( Fig. 7a ), initial pyrite mineralization must occur rapidly to circumvent compression, and must continue to fill the entire volume of the organism. If full pyritization occurs entirely in the BSR zone, then the decaying carcass must stay in the BSR zone for a sufficient amount of time, requiring a thick BSR zone and/or a slow sedimentation rate following burial. The initial smothering event that entrapped the Conotubus organism rapidly placed it below the oxic zone of aggressive aerobic decay, and subsequent sedimentation proceeded sufficiently slowly to ensure a long enough duration in the BSR zone for complete pyritization. This scenario is consistent with the δ 34 S PY data, with greater outer-edge values suggesting an initial period of relatively rapid BSR, ensuring three-dimensional structural integrity, followed by a progressive decrease in BSR rate ( Supplementary Fig. 1 ) accompanying greater isotopic fractionation and lower δ 34 S PY values. Volumetric considerations, however, suggest a shortage of organic fuel from the Conotubus soft-tissue itself, which would require either an exogenous source of carbon or production of de novo organic carbon within the organic nucleus (for instance, by in situ chemoautotrophs) to continue fuelling further sulfide production once the labile soft tissues of Conotubus were exhausted. Alternatively, pyritization could continue in the methanogenesis zone where BSR is disfavoured but residual or downward-diffusing porewater HS – (or Fe–S complexes [47] ) support pyrite overgrowth and continued pyritization. This extended period of overgrowth may not show any clear textural change, but would obscure the anticipated U-shaped δ 34 S PY profile because residual porewater HS – tends to have greater δ 34 S values. In combination, the observed subtle textural variations ( Fig. 2b,c ) and higher δ 34 S PY values along millimetric crystal edges may support this alternative scenario. Regardless, the keys for complete pyritization are rapid burial and initial pyritization to maintain structural integrity, followed by prolonged pyrite overgrowth within and perhaps below a relatively thick BSR zone to completely fill Conotubus tubes with pyrite. Incomplete but three-dimensional pyritization ( Fig. 7b ) requires the same facilitating taphonomic conditions as complete pyritization, including rapid placement in the BSR zone and initiation of pyritization to maintain three-dimensionality, but instead experiences closure of the pyritization process before complete infilling of the Conotubus tube with pyrite. As such, temporal limitation of one or more of the required chemical components, such as diffusive extinction of sulfate, may limit the extent of the BSR zone. With or without BSR zone restriction, the decaying Conotubus organism is likely pushed down into the methanogenesis zone due to high post-burial sedimentation rate, such that pyritization in the BSR zone is prematurely terminated. Alternatively, these incompletely pyritized tubes may persist within the BSR zone, but with cessation of pyritization due to exhaustion of metabolizable organic material and a shortage of exogenous carbon input. The interior space originally occupied by the Conotubus animal then becomes a central void, which is subsequently infilled with carbonate cements. The timing of carbonate cementation may depend on the electron donor used in BSR ( Supplementary Table 3 ). Two scenarios are plausible: (1) the BSR respiration pathway does not produce acidity and carbonate cementation is synchronous with pyritization; or (2) carbonate cementation follows dissipation of a lower pH microenvironment generated with BSR production of acidity. In either case, no organic material remains or at least none is preserved through kerogenization. Regardless of which alternative is more realistic, the true preservational distinction between complete and incomplete three-dimensional pyritization hinges on the duration, not the initiation, of pyrite formation. With regard to complete pyritization, we suggest that continuing pyrite overgrowth is necessary for complete Conotubus tube infill, whereas incompletely pyritized tubes instead are infilled with carbonate cements after premature termination of pyritization. At the other end of the Gaojiashan preservational spectrum are kerogenized carbonaceous compressions. While models for kerogenization invoke the same facilitating taphonomic conditions for pyritization, three-dimensional structural rigidity is not preserved, and instead organic tissues are stabilized to form geologically robust but two-dimensionally compressed carbonaceous remains. In the kerogenization taphonomic modes, pyritization is necessarily limited for tissues to be preserved as carbonaceous compressions. The potential key is a rapid post-burial sedimentation rate and/or a narrower BSR zone, such that the fossilizing Conotubus tube is much more quickly moved through the BSR zone with little pyritization, thus positioning the decaying organism within the methanogenesis zone shortly following the onset of decay. In such a case, Conotubus tubes that exhibit an appreciable amount of pyritization ( Fig. 7c ) may have stayed in the BSR zone long enough to facilitate localized pyritization but not extensively sustained for pyritization to maintain three-dimensional structural integrity. Kerogenized Conotubus with only diffuse pyrite ( Fig. 7d ) likely experience the majority of preservation within the methanogenesis zone during the earliest stages of decay, thus spending only very limited time in the BSR zone due to a high post-burial sedimentation rate and/or a narrowed BSR zone. Following these conditions, the fossil is predominantly comprised of carbonaceous remains from kerogenization within the methanogenesis zone. Methanogens are incapable of decomposing higher molecular weight organic compounds, commonly using acetate as the terminal electron acceptor [48] (generalized: CH 3 COO – +H 2 O→CH 4 +HCO 3 – ). If the breakdown of high-molecular weight compounds via bacterial fermentation (generalized: C 6 H 12 O 6 +4 H 2 O→2 CH 3 COO – +2 HCO 3 – +4 H + +4 H 2 ) is mostly limited to metabolically labile tissues, and aggressive aerobic degradation (generalized: CH 3 COO – +O 2 →2 CO 2 +H 2 O+OH – ) [48] was limited as a result of rapid burial, only the most recalcitrant structures such as the Conotubus tube walls will enter the fossil record. A few alternative scenarios should also be considered. First, the Conotubus remains may indeed undergo degradation within the BSR zone, but instead occupy microenvironments that are substantially limited in either or both reactive iron or sulfate thus hindering pyrite precipitation. Second, the invocation of minimal ambient organic material [13] for pyritization may not hold in cases of kerogenization. That is, SRB may prefer disseminated organic sources if Conotubus is emplaced within comparatively more organic-rich sediments, with Conotubus thus avoiding BSR-degradation and localized pyritization. Regardless, in either case, organic degradation is clearly limited to labile tissues, such that only the recalcitrant tissues are eventually preserved as kerogens. Previous biostratinomical analysis of the late Ediacaran Gaojiashan Lagerstätte has established that event deposits played an important role in the preservation of Gaojiashan fossils [11] , but the post-burial mineralization processes leading to the observed pyritization–kerogenization gradient of preservation remain elusive. On the basis of geochemical analyses of three-dimensionally pyritized Conotubus specimens, we have established that the pyritization process proceeded centripetally from a rim of micrometric pyrite nucleated on the tube wall and fuelled by SRB degradation of labile tissues within the tube. This process can be described using a diffusion–precipitation model [31] , [32] , modified to account for the role of an organic tube in promoting the onset of pyritization by providing a preferable substrate for nucleation. We suggest that preservation along the pyritization–kerogenization gradient can be understood as variations in the placement and duration of the carcass within the BSR and methanogenesis zones. The amount of time spent in each zone is principally influenced by post-burial sedimentation rate and/or BSR zone thickness, the latter of which is also related to the availability of metabolizable organic material and sulfate. The fossils that show three-dimensional pyritization, whether pervasive or incomplete, spend more time in the BSR zone. In contrast, those that are two-dimensional carbonaceous compressions, either with extensive or diffuse pyrite association, are more rapidly buried in the methanogenesis zone. In each case, degradation is required for preservation, and each mode may be viewed as a complex balance between decay and mineralization. These preservation processes, whether pyritization or kerogenization, are governed by the same suite of facilitating taphonomic conditions, are primarily influenced by microbial decay pathways, and differ principally in the duration of interactions with the BSR and methanogenesis zones. Thus, the scientific conversation regarding contributing factors of Beecher’s Trilobite-type pyritization and Burgess Shale-type carbonaceous compression should be shifted from facilitating factors such as a lack of bioturbation [49] , [50] and bed-capping carbonate cements [18] , to those that drive mineralization and stabilization processes and are directly responsible for fossil preservation. Materials The Conotubus hemiannulatus specimens examined in this study were collected from the Gaojiashan Member of the Dengying Formation at Gaojiashan in Ningqiang county, southern Shaanxi Province, South China [28] . Located in the northwest margin of the Yangtze Platform ( Supplementary Fig. 2A ), the Gaojiashan region has numerous exposures of Ediacaran–Cambrian strata with broadly similar stratigraphy (from lower to upper): siliciclastic-dominated Doushantuo Formation; dolostone-dominated Dengying Formation; and phosphorite and carbonate of the basal Cambrian Kuanchuanpu Formation. The Dengying Formation is tripartite ( Supplementary Fig. 2B ), consisting of (from lower to upper): thick-bedded, vuggy, peritidal dolostones of the ~300-m-thick Algal Dolomite Member; thin-bedded calcareous siltstones, mudstones and limestones of the ~55-m-thick Gaojiashan Member that hosts the Gaojiashan Lagerstätte; and thick-bedded, vuggy, microbially laminated-to-stromatolitic, peritidal dolostone of the ~200-m-thick Beiwan Member. Correlation with the radiometrically dated Dengying Formation in the Yangtze Gorges suggests that the Gaojiashan Lagerstätte is constrained between 551 and 541 Myr ago [51] , [52] . Gaojiashan fossils mostly occur within millimetric beds of fine-grained calcisiltite-siltstone of the Gaojiashan Member, interpreted to have been deposited below storm wave base. Biostratinomic analysis of the Gaojiashan biota indicates that rapid event deposition played a key role in the exceptional preservation of Gaojiashan fossils [11] . The Gaojiashan biota is dominated by weakly biomineralized to non-biomineralized tubular and ribbon-like fossils (for example, Cloudina , Conotubus , Gaojiashania , Shaanxilithes and Sinotubulites ), and also includes protolagenid microfossils, algal debris, ichnofossils and microbial mat textures [11] , [28] , [53] , [54] , [55] , [56] , [57] , [58] , [59] . The focus of this study, Conotubus hemiannulatus , is currently only known from the Gaojiashan Lagerstätte. Showing similarities in construction ( Fig. 1d ) and epibenthic life-mode, Conotubus has been interpreted as a possible evolutionary precursor of Cloudina [28] , [55] . Conotubus differs from Cloudina in its tube composition, as Conotubus was likely only weakly biomineralized at most [28] . The fossiliferous unit occurs ~18–49 m above the base of the Gaojiashan Member, with the Conotubus –dominated biofacies within the 26–39 m range corresponding to positive δ 13 C and negative δ 18 O excursions [60] . Rare earth elemental geochemistry [60] suggests that the Gaojiashan Member was deposited in a restricted shallow sea environment, with riverine influx, common storm deposition influence [11] , and high bioproductivity. The samples studied herein were collected from calcareous siltstones 28–45 m above the base of the Gaojiashan Member ( Supplementary Fig. 2B ). Three pyritized Conotubus hemiannulatus specimens, collected 28–29 m above the base of the Gaojiashan Member ( ★ 1 in Supplementary Fig. 2B ), were trimmed to sub-25-mm pieces, vacuum embedded in low-viscosity epoxy, and then ground and polished to make two longitudinal cross-sections and one transverse cross-section. These three specimens (reposited at the University of Missouri, Columbia; specimen numbers: GJS-Cono001 to GJS-Cono003) were imaged and compositionally analysed using scanning electron microscopy (SEM)/energy-dispersive X-ray spectroscopy (EDS). Sulfur isotopic compositions of pyrite (δ 34 S PY , reported as ‰-VCDT) were measured in situ using SIMS and on microdrilled powders using IRMS. A fourth specimen, collected at 37–38 m above the base of the Gaojiashan Member ( ★ 3 in Supplementary Fig. 2B ), on a larger slab was polished to make a transverse cross-section. This specimen (reposited at the Virginia Tech; specimen number: 1GH2-70A) was analysed using SEM/EDS, ultraviolet photoluminescence microscopy and in situ X-ray diffraction (XRD). Both specimen number 1GH-70A and a non-fossiliferous slab, collected at 44–45 m above the base of the Gaojiashan Member ( ★ 4 in Supplementary Fig. 2B ), were microdrilled for IRMS δ 13 C and δ 18 O analyses (see Fig. 6a,b for drilling maps). An additional slab, collected 32 m above the base of the Gaojiashan Member ( ★ 2 in Supplementary Fig. 2B ), was analysed via IRMS for δ 34 S CAS (data reported in Supplementary Table 1 ). Scanning electron microscopy All SEM and EDS analyses ( Fig. 2a–c,g; and Fig ; Fig. 4a,b,e–g ; Fig. 5b,e,f ) were conducted using an FEI company Quanta 600 field-emission variable-pressure SEM with an integrated Bruker AXS Quantax 400 high-speed silicon-drift EDS detector (Virginia Tech Institute for Critical Technology and Applied Science Nanoscale Characterization and Fabrication Laboratory). The specimens were analysed in high-vacuum mode (~6 × 10 −6 Torr), ~10 mm working distance, 20 keV beam accelerating voltage, 5.0 spot size (approximation of beam diameter and specimen current) and a system take-off angle of 35° for EDS analyses. EDS point scans were conducted for 100 s live-time, and elemental maps were collected for 600 s live-time. Secondary ion mass spectroscopy All SIMS analyses followed δ 34 S PY methods described in ref. 32 , using a Cameca 7f GEO magnetic sector system (Virginia Tech Institute for Critical Technology and Applied Science Nanoscale Characterization and Fabrication Laboratory). A Cs + primary beam with 1 nA current at an energy of 20 kV was used to sputter the specimen, and the 32 S and 34 S isotopes were detected using dual Faraday cup detectors from a ~10 μm analytical spot. Mass resolution of ~2,000 m per Δm was used to resolve the 32 S from 16 O 2 mass interference. A total of 214 spots across three specimens were analysed ( Supplementary Table 1 ; Figs 2a,d–f ; Fig. 3a,b ; Fig. 4b–d ), and measured δ 34 S PY values are reported as ‰ deviation from VCDT (Vienna Cañon Diablo Troilite; 34 S/ 32 S=0.0450045 ref. 61 ) calibrated via a Balmat pyrite standard (δ 34 S Balmat =15.1‰-VCDT; 34 S/ 32 S=0.04568407 refs 62 , 63 ). Each SIMS spot measurement consisted of 10 cycles of 34 S/ 32 S ratios acquired from the same physical spot after ~2-min presputter to remove potential surface contamination. The duration of individual spot analyses was ~5 min, not including presputter. One-sigma errors of sample δ 34 S PY measurements were calculated from the instrumental standard error report of the 10 cycles, converted to ‰-VCDT. Ultraviolet photoluminescence and X-ray diffraction Photoluminescence microscopy and in situ XRD analyses were conducted on a UV microscope (Olympus BX51) and a Rigaku Rapid II X-ray diffraction system with a 2D image plate, in the S.W. Bailey X-ray Diffraction Laboratory, Department of Geoscience, University of Wisconsin. The polished cross-sectional slab of Conotubus , specimen number 1GH2-70A, was used in the analyses. All diffraction patterns were collected using reflection mode. Single-crystal diffraction patterns were also obtained to understand the crystallographic relationship between the dolomite and calcite in the zoned crystals ( Fig. 5c,d,g ). Isotope ratio mass spectroscopy Carbon and oxygen IRMS analyses were carried out at the University of Maryland and the Northwest University in Xi’an. Approximately 100 μg microdrilled powder was allowed to react for 10 min at 90 °C with anhydrous H 3 PO 4 in a Multiprep inlet system connected to an Elementar Isoprime dual inlet mass spectrometer for δ 13 C and δ 18 O analysis. Isotopic results are expressed in the standard δ notation as ‰ deviation from VPDB. Uncertainties determined by multiple measurements of NBS-19 were better than 0.05‰ (1σ) for both C and O isotopes. Carbonate-associated sulfate sulfur IRMS analysis was carried out at Indiana University. After trimming to remove visible veins and weathering rinds and ultrasonically cleaning in distilled deionized water, 56.3 g of whole rock was crushed and pulverized into powder of <200 mesh size (74 μm) using a split-discus mill. Sulfate extraction followed the recommended protocol of ref. 64 . Ultra-pure Milli-Q water (18 MΩ), purified NaCl, and distilled HCl were used to create solutions for leaching and acid digestion of the sample. The powder was immersed in 10% NaCl solution under constant magnetic stirring at room temperature until no sulfate was present in filtrate solutions. After water-leaching steps, the carbonate sample was dissolved in 10‰ HCl solution. The slurry was decanted and vacuum filtered through a 0.45-μm cellulose membrane filter. The acid-leached sulfate was collected as BaSO 4 by adding saturated BaCl 2 solution. All collected BaSO 4 samples were further purified by the DDARP method of ref. 65 . BaSO 4 was converted to SO 2 using an Elemental Analyzer at 990 °C and the δ 34 S CAS measurement was conducted on a Thermo-Electron Delta V Advantage mass spectrometer in continuous-flow mode. In addition, pyrite from samples GJS-Cono001 to GJS-Cono003 was microdrilled and analysed for δ 34 S PY (s.d.=±0.3‰) to compare with SIMS results. Pyrite extraction followed the chromium reduction method of ref. 66 . Sulfur isotopic results are expressed in the standard δ notation as ‰ deviation from VCDT. How to cite this article: Schiffbauer, J. D. et al . A unifying model for Neoproterozoic–Palaeozoic exceptional fossil preservation through pyritization and carbonaceous compression. Nat. Commun. 5:5754 doi: 10.1038/ncomms6754 (2014).